Synergistic geometric and electronic effects for electrochemical reduction of carbon dioxide using gold–copper bimetallic nanoparticles Highly efficient and selective electrochemical reduction of carbon dioxide represents one of the biggest scientific challenges in artificial photosynthesis, where carbon dioxide and water are converted into chemical fuels from solar energy. However, our fundamental understanding of the reaction is still limited and we do not have the capability to design an outstanding catalyst with great activity and selectivity a priori . Here we assemble uniform gold–copper bimetallic nanoparticles with different compositions into ordered monolayers, which serve as a well-defined platform to understand their fundamental catalytic activity in carbon dioxide reduction. We find that two important factors related to intermediate binding, the electronic effect and the geometric effect, dictate the activity of gold–copper bimetallic nanoparticles. These nanoparticle monolayers also show great mass activities, outperforming conventional carbon dioxide reduction catalysts. The insights gained through this study may serve as a foundation for designing better carbon dioxide electrochemical reduction catalysts. Energy and environmental problems represent one of the greatest challenges facing mankind in this century. Despite tremendous efforts to develop renewable energy sources [1] , [2] , [3] , [4] , [5] , [6] , [7] , still the majority of energy used is derived from non-renewable fossil fuels. One attractive option to solve this problem is the electrochemical reduction of carbon dioxide into fuels [8] . Reducing carbon dioxide, an abundant carbon source, into value-added fuels using a renewable energy input (that is, artificial photosynthesis) would allow us to reduce our dependence on conventional fossil fuels, mitigate CO 2 emissions and make our society more sustainable. Furthermore, chemical fuels produced from carbon dioxide could be readily implemented in the current energy infrastructure, allowing a quick and smooth transition towards a renewable energy society. However, fundamental scientific challenges remain for the basic understanding of electrochemical carbon dioxide reduction process, which limit our capability of rationally designing high-performance CO 2 reduction catalysts. The CO 2 reduction reaction itself is much more complex than the related hydrogen evolution (HER) or oxygen evolution reaction (OER), as multiple electron and proton coupling steps are typically involved in several different reaction pathways, leading to many possible final products [9] , [10] . In addition, most of the materials studied as CO 2 reduction catalysts to date require large over-potentials and typically are also active for HER [11] , [12] , which results in low turnover rates (TOR) to CO 2 reduction products at moderate over-potentials. Furthermore, there is an additional issue of catalyst deactivation, which must be addressed for sustained production of fuels from CO 2 (refs 9 , 13 ). Despite the limitations on the fundamental understanding of electrochemical reduction of CO 2 , there have been great efforts in the past few decades to address this issue either experimentally [8] , [9] , [10] , [11] , [12] , [13] , [14] , [15] , [16] , [17] , [18] , [19] or theoretically [20] , [21] , [22] . A wide variety of metal electrodes have been examined [9] as CO 2 reduction catalysts with a focus on Cu [10] , [11] , [14] , [15] , [18] , Au [16] , [23] and Sn [17] , as other metals are mostly inactive. In particular, Cu has gained the most interest because of its capability to reduce CO 2 into hydrocarbon fuels, such as methane or ethylene. Even though some progress has been made for these catalysts in terms of increasing TOR and reducing over-potentials, there is still much to be learned to develop a better understanding of the reaction and the principles required to design an efficient catalyst. More recently, one approach that has been suggested to enhance the catalytic activity and selectivity for CO 2 reduction is alloying [21] , [22] . By alloying, it is believed that we might be able to tune the binding strength of intermediates on a catalyst surface to enhance the reaction kinetics for CO 2 reduction. Nanoparticles provide an ideal platform for studying this effect. Through appropriate synthetic processes, a wide range of compositions, sizes and shapes can be accessed, allowing for deeper understanding of catalyst performance through precise control of active sites [24] . Furthermore, nanoparticles have high surface-to-volume and surface-to-mass ratio, which are advantageous for achieving high mass activity [23] , [24] . For this reason, we use Au–Cu bimetallic nanoparticles in a monolayer platform to study their CO 2 reduction activity. Using this monolayer platform, we are able to quantitatively compare activity and selectivity as a function of Au and Cu composition. Moreover, we can achieve efficient catalyst loading, resulting in a significant enhancement in its mass activity. Insights gained through this quantitative comparison will help to develop design principles for high-performance CO 2 reduction catalysts. Characterization of Au–Cu bimetallic nanoparticle catalysts The Au–Cu bimetallic system has been suggested as a potential CO 2 reduction catalyst in previous reports [25] , [26] . However, there has not been a systematic study to precisely understand its activity as function of its composition. Furthermore, Au and Cu have been identified to possess intermediate binding strength favourable for CO 2 reduction [21] , [22] ; hence, they serve as a good starting point to tune the energetics of the intermediate binding to achieve even higher activity. 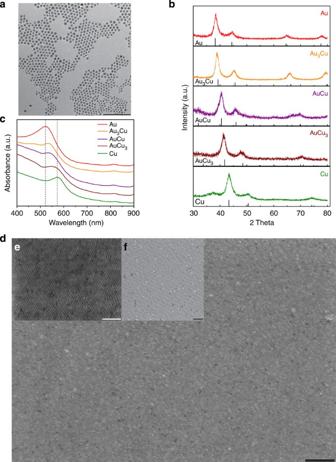Figure 1: Characterization and assembly of Au–Cu bimetallic nanoparticles. (a) TEM image of AuCu3nanoparticles (scale bar, 100 nm). Average size 11.20±1.65 nm. (b) XRD patterns of Au–Cu bimetallic nanoparticles compared with diffraction patterns from the database (Au, JCPDS 03-065-2870; Au3Cu, JCPDS 01-071-5023; AuCu, JCPDS 00-025-1220; AuCu3, JCPDS 03-065-3249; Cu, JCPDS 00-004-0836). A small peak at 2θ ~37° in the XRD pattern of Cu indicates the presence of a Cu2O shell. (c) Ultraviolet–visible spectra of Au–Cu bimetallic nanoparticles. Dotted lines indicate the SPR peak of pure Au (~523 nm) and Cu (~570 nm) nanoparticles. (d) Scanning electron microscopy (SEM) image of a AuCu3nanoparticle monolayer transferred to a substrate using Langmuir–Schaefer technique (scale bar, 200 nm). (e) Inset figure with a higher-magnification SEM image of a Au3Cu nanoparticle monolayer (scale bar, 100 nm). (f) Inset figure with a TEM image of a Cu nanoparticle monolayer transferred to a TEM grid (scale bar, 100 nm). Figure 1a is a transmission electron microscopy (TEM) image of AuCu 3 nanocrystals as synthesized. The synthetic procedures were modified from the methods reported previously [27] . Nanoparticles with different stoichiometric ratios of Au-to-Cu (Au, Au 3 Cu, AuCu, AuCu 3 and Cu) were synthesized in a similar manner with average size all close to 10~11 nm ( Supplementary Figs 1 and 2 ), so that once assembled in a monolayer the catalytically active surface area for each electrode is essentially identical. The composition of each nanoparticle is confirmed using a number of methods. X-ray diffractometry (XRD) shows that the XRD pattern of each particle ( Fig. 1b ) matches with the corresponding characteristic patterns of each phase, although we find Cu to inevitably have a thin oxide shell, as can be seen from its XRD data [28] . In addition, Au and Cu atoms are randomly distributed within the lattice, which is expected considering the synthetic conditions [29] . Ultraviolet-visible spectroscopy is also a useful way to characterize nanoparticles. Au and Cu nanoparticles in their pure phase exhibit characteristic surface plasmon resonance (SPR) peaks at ~523 and ~570 nm (refs 26 , 30 , 31 ). As the content of Cu increases in a pure Au nanoparticle by forming an alloy, the SPR peak of Au red-shifts towards the SPR peak of Cu with some broadening [26] , [30] ( Fig. 1c ). The SPR peaks (λ SPR =533 nm for Au 3 Cu, 539 nm for AuCu and 549 nm for AuCu 3 ) also match well with their composition [26] , [30] . Energy-dispersive X-ray spectroscopy was further used to confirm the composition of the nanoparticles ( Supplementary Fig. 3 ). All these results confirmed that we have synthesized monodisperse Au–Cu bimetallic nanoparticles with specific stoichiometric ratios of Au-to-Cu. Figure 1: Characterization and assembly of Au–Cu bimetallic nanoparticles. ( a ) TEM image of AuCu 3 nanoparticles (scale bar, 100 nm). Average size 11.20±1.65 nm. ( b ) XRD patterns of Au–Cu bimetallic nanoparticles compared with diffraction patterns from the database (Au, JCPDS 03-065-2870; Au 3 Cu, JCPDS 01-071-5023; AuCu, JCPDS 00-025-1220; AuCu 3 , JCPDS 03-065-3249; Cu, JCPDS 00-004-0836). A small peak at 2θ ~37° in the XRD pattern of Cu indicates the presence of a Cu 2 O shell. ( c ) Ultraviolet–visible spectra of Au–Cu bimetallic nanoparticles. Dotted lines indicate the SPR peak of pure Au (~523 nm) and Cu (~570 nm) nanoparticles. ( d ) Scanning electron microscopy (SEM) image of a AuCu 3 nanoparticle monolayer transferred to a substrate using Langmuir–Schaefer technique (scale bar, 200 nm). ( e ) Inset figure with a higher-magnification SEM image of a Au 3 Cu nanoparticle monolayer (scale bar, 100 nm). ( f ) Inset figure with a TEM image of a Cu nanoparticle monolayer transferred to a TEM grid (scale bar, 100 nm). Full size image Nanoparticle assembly (or self-assembly) has been the subject of research for use of these unique structures in a wide variety of applications [32] , [33] , [34] , [35] , [36] , [37] . Among several approaches that lead to monolayer assemblies, we implemented the solvent evaporation-mediated self-assembly approach modified from its original method [38] , to fabricate nanoparticle monolayer platforms. Once assembled, the nanoparticle monolayers were transferred onto a glassy carbon substrate using the Langmuir–Schaefer method and tested in our electrochemical setup for CO 2 reduction. Figure 1d shows a scanning electron microscopy image of a AuCu 3 monolayer on a substrate. Most of the area is covered with the nanoparticle monolayer with high degree of ordering throughout the substrate, although it also contains some defective spots such as vacancies. CO 2 reduction activity of Au–Cu bimetallic nanoparticles To quantitatively determine and compare catalytic activity, the monolayered nanoparticles were analysed in our custom-designed electrochemical setup coupled with gas chromatography. The effluent gas from the electrochemical cell went through the sampling system of the gas chromatography and gas products were analysed in real-time, while the liquid products were analysed after the reaction by quantitative nuclear magnetic resonance spectroscopy. Electrolysis was performed under standard conditions of 0.1 M KHCO 3 electrolyte saturated with CO 2 . 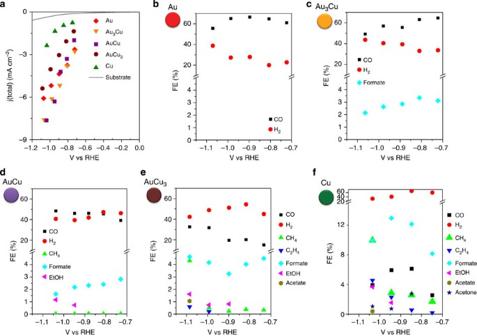Figure 2: Catalytic activities of Au–Cu bimetallic nanoparticles. (a) Total current density plot of Au–Cu bimetallic nanoparticles. Current density is from the geometric area of the electrodes. All measurements were under the same environment of 0.1 M KHCO3(pH 6.8) at 1 atm CO2and room temperature. The grey line indicates the activity of the bare substrate from linear sweep voltammetry (50 mV s−1) stabilized after multiple cycles. For the nanoparticles, the current density is averaged for the first 5 min of each run to rule out any effects that mask their fundamental activity such as extensive bubble formation. On the plot is the average current density of multiple runs at each potential. SeeSupplementary Figs 4 and 5. (b) FE for each product of Au. (c) Au3Cu. (d) AuCu. (e) AuCu3. (f) Cu. Other minor products were identified, such as methanol, acetaldehyde and glycoaldehyde with nanoparticles of higher Cu content, although not quantified. SeeSupplementary Table 1. Figure 2a shows the overall activity of the Au–Cu bimetallic nanoparticles under identical reaction conditions ( Supplementary Figs 4 and 5 ). Pure Cu nanoparticles exhibit the lowest overall activity, while increasing the Au content enhances the activity up to the point where Au 3 Cu seems to exhibit the highest activity among the series. However, as the overall current density also includes the current from HER, it is difficult to determine which catalyst performs better for CO 2 reduction just from this plot. Furthermore, as electrochemical CO 2 reduction typically leads to a large number of chemical products, the overall current must be divided into individual products to get a quantitative understanding of the activity and selectivity as function of composition. Figure 2: Catalytic activities of Au–Cu bimetallic nanoparticles. ( a ) Total current density plot of Au–Cu bimetallic nanoparticles. Current density is from the geometric area of the electrodes. All measurements were under the same environment of 0.1 M KHCO 3 (pH 6.8) at 1 atm CO 2 and room temperature. The grey line indicates the activity of the bare substrate from linear sweep voltammetry (50 mV s −1 ) stabilized after multiple cycles. For the nanoparticles, the current density is averaged for the first 5 min of each run to rule out any effects that mask their fundamental activity such as extensive bubble formation. On the plot is the average current density of multiple runs at each potential. See Supplementary Figs 4 and 5 . ( b ) FE for each product of Au. ( c ) Au 3 Cu. ( d ) AuCu. ( e ) AuCu 3 . ( f ) Cu. Other minor products were identified, such as methanol, acetaldehyde and glycoaldehyde with nanoparticles of higher Cu content, although not quantified. See Supplementary Table 1 . Full size image One way of doing this is to examine the Faradaic efficiencies (FE) for each product, which are shown in Fig. 2b–f . The results are interesting, as it is generally believed Cu is the only catalyst capable to produce a wide range of products [10] , [14] , [18] . Not only do the Au–Cu bimetallic nanoparticles make products usually seen on Cu, but the FE of these products shifts as the composition is changed ( Supplementary Table 1 ). As the Cu content increases, the total number of products increases and the pure Cu nanoparticles exhibit the largest number in product type. Among the products that require more than two electron transfers, methane and ethylene are considered as major products that can be produced from Cu [10] , [11] . For methane and ethylene, the FE decreases substantially as more Au gets incorporated into the nanoparticle, eventually leading to a total loss of these products for nanoparticles with high concentrations of Au. Further, Fig. 2b–f reveals that the trends in FE for CO and H 2 are opposite as the composition shifts. FE for CO increases with Au content, while FE for H 2 decreases as the Au content increases. For pure Au nanoparticles, the FE for CO is close to ~65%, which is consistent with other reports for Au nanoparticles of similar size [23] . In the case of formate, which is known as the largest molecular liquid product from Cu, the trend seems to follow hydrocarbon species such as methane, although the decrease is not drastic. Based on this analysis and comparison, the reactions that require a hydrogen atom binding to the carbon along the reaction pathway tend to have decreased in FE for their final products following the same trend for H 2 , while FE of CO shows the opposite trend where protonation happens at the hydroxyl end group of a carboxyl intermediate stabilized on the surface [20] , [21] , [22] . To protonate the carbon atom, a surface-stabilized proton has to be near the active site and this indicates that the product distribution in CO 2 reduction might be related to the binding strength of hydrogen on the surface of a catalyst. In principle, we could expect that the binding strength of all the intermediates that occur along the reaction pathway would govern the activity/selectivity, as it determines the interaction of the intermediates with the catalyst and lead into different reactions pathways and final chemical products. Therefore, at this point, it is reasonable to assume that by tuning the composition of Au–Cu bimetallic nanoparticles, we are tuning the degree of stabilization of the intermediates on these nanoparticle surfaces, and consequently, different final chemical product profiles were observed. 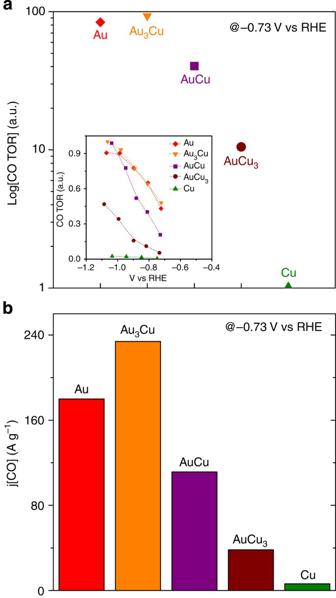Figure 3: Trends in TORs of Au–Cu bimetallic nanoparticles and their mass activity. (a) Relative TORs for carbon monoxide compared at ~−0.73 V vs RHE. TOR calculations are based on the partial current density and the TOR of Cu is set to one. Each data point is spaced equally apart on thexaxis and the TORs are plotted in log scale. Potential is chosen to minimize any mass transport effects. Inset shows relative CO TOR (where all the data are normalized to the highest value) as a function of potential. SeeSupplementary Fig. 6for other products. (b) CO mass activity of Au–Cu bimetallic nanoparticles at ~−0.73 V vs RHE. Mass activity is based on the overall mass of Au and Cu. SeeSupplementary Fig. 10andSupplementary Table 2. Figure 3a compares the relative TOR for CO at −0.73 V versus reversible hydrogen electrode (RHE) for these nanoparticles with different compositions ( Supplementary Fig. 6 ). We found that the activity follows a volcano shape with a peak activity for Au 3 Cu (Au 3 Cu~93.1 times, Au~83.7 times and AuCu~40.4 times higher relative to Cu). This trend can be understood by considering the elementary reaction steps from CO 2 to CO [22] . In this reaction, CO 2 is adsorbed onto the surface as COOH and further reduced to CO. Therefore, the binding strength of COOH and CO essentially governs CO TOR. To enhance the CO production kinetics, a catalyst has to stabilize COOH more strongly relative to CO [22] , so that CO 2 readily activates to COOH and desorbs as CO. However, this is difficult to achieve with a monometallic catalyst because of the scaling relation, which shows that the binding strengths of different intermediates scale together [21] , [39] . Alloy catalysts, on the other hand, could potentially stabilize COOH relative to CO by forming an additional bond at the oxygen end with an oxophilic element (that is, Cu) on the catalyst surface [21] , [22] . Based on this observation, the CO activity of Au–Cu bimetallic nanoparticles can be explained in terms of (1) the electronic effect where the binding of intermediates can be tuned using different surface composition and (2) the geometric effect that has to do with the local atomic arrangement at the active site, which allows the catalyst to deviate from the scaling relation. Figure 3: Trends in TORs of Au–Cu bimetallic nanoparticles and their mass activity. ( a ) Relative TORs for carbon monoxide compared at ~−0.73 V vs RHE. TOR calculations are based on the partial current density and the TOR of Cu is set to one. Each data point is spaced equally apart on the x axis and the TORs are plotted in log scale. Potential is chosen to minimize any mass transport effects. Inset shows relative CO TOR (where all the data are normalized to the highest value) as a function of potential. See Supplementary Fig. 6 for other products. ( b ) CO mass activity of Au–Cu bimetallic nanoparticles at ~−0.73 V vs RHE. Mass activity is based on the overall mass of Au and Cu. See Supplementary Fig. 10 and Supplementary Table 2 . Full size image The electronic effect on the binding strength of intermediates is due to the change in the electronic structure of a catalyst. For transition metals, the way their d -band interacts with the adsorbate determines the binding strength. The trend is that the more low lying (relative to the Fermi level) the d -band, the weaker the binding due to the occupancy of anti-bonding states [39] . 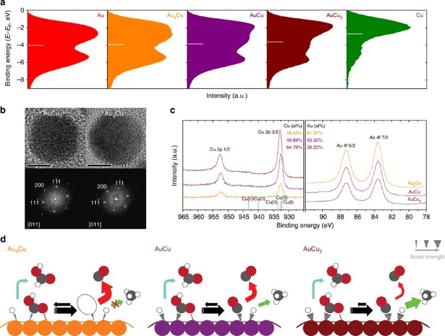Figure 4: Structural characterization of Au–Cu bimetallic nanoparticles. (a) Surface valence band photoemission spectra of Au–Cu bimetallic nanoparticles. All the spectra are background corrected. The white bar indicates its centre of gravity. For comparison, the upper limit of integration is fixed to −9.0 eV in binding energy. (b) High-resolution transmission electron microscopy image of AuCu3and Au3Cu, and their fast fourier transform. Scale bar, 5 nm. (c) X-ray photoemission spectra at grazing angle (85°) on Au–Cu bimetallic nanoparticle monolayers. SeeSupplementary Fig. 8for the survey spectra. (d) Schematic showing the proposed mechanism for CO2reduction on the catalyst surface of Au–Cu bimetallic nanoparticles. Filled circles with grey is C, red is O and white is H. The relative intermediate binding strength is indicated by the stroke weight (on the top right corner). Additional binding between the COOH and the catalyst surface is presented as a dotted line. Arrows between the adsorbed COOH and adsorbed CO is to show the difference in probability of having COOH adsorbed on different types of surfaces. Coloured arrows indicate the pathway to each product: red for CO, blue for formate and green for hydrocarbons. Larger arrows indicate higher turnover. Figure 4a is the surface valance band spectra of Au–Cu bimetallic nanoparticles collected by high-resolution X-ray photoemission spectroscopy (XPS) on the nanoparticle monolayers. Using Al Kα source, the binding energy was scanned from 0 to 20 eV and each spectrum was collected over ~1,000 scans. The spectra reveal that the d -band and its centre of gravity gradually shift downwards from Cu to Au [40] . According to this trend, the binding strength for COOH and CO, which is mainly from the bond between the active site and the carbon, should decrease as Au content increases. Then the binding strength to Au–Cu bimetallic nanoparticles would lie in between Au and Cu following the scaling trend, which can also be estimated from the interpolation principle [39] . It is known that Au has the optimum binding strength for COOH and CO to reach peak activity among the transition metal catalysts for CO 2 to CO conversion [22] . Therefore, from the electronic effect, Au is expected to be at the peak of the volcano, while the activity scales down linearly to Cu as the composition shifts. However, we observe peak activity for Au 3 Cu and also activities higher for AuCu and AuCu 3 than predicted from a trendline between Au and Cu. In addition to the interesting trend in CO activity, the shift in selectivity and the presence of formate produced from Au 3 Cu but not pure Au needs to be understood from more than the electronic effect, considering the similar electronic structures of Au and Au 3 Cu. These observations indicate that the activity is not solely determined from the electronic effect. Figure 4: Structural characterization of Au–Cu bimetallic nanoparticles. ( a ) Surface valence band photoemission spectra of Au–Cu bimetallic nanoparticles. All the spectra are background corrected. The white bar indicates its centre of gravity. For comparison, the upper limit of integration is fixed to −9.0 eV in binding energy. ( b ) High-resolution transmission electron microscopy image of AuCu 3 and Au 3 Cu, and their fast fourier transform. Scale bar, 5 nm. ( c ) X-ray photoemission spectra at grazing angle (85°) on Au–Cu bimetallic nanoparticle monolayers. See Supplementary Fig. 8 for the survey spectra. ( d ) Schematic showing the proposed mechanism for CO 2 reduction on the catalyst surface of Au–Cu bimetallic nanoparticles. Filled circles with grey is C, red is O and white is H. The relative intermediate binding strength is indicated by the stroke weight (on the top right corner). Additional binding between the COOH and the catalyst surface is presented as a dotted line. Arrows between the adsorbed COOH and adsorbed CO is to show the difference in probability of having COOH adsorbed on different types of surfaces. Coloured arrows indicate the pathway to each product: red for CO, blue for formate and green for hydrocarbons. Larger arrows indicate higher turnover. Full size image The geometric effect also plays an important role in determining catalytic activity, as it has to do with the atomic arrangement at the active site. The way the active site is configured can have a large effect on the binding strength of intermediates [41] . In the case of Au–Cu bimetallic nanoparticles, further stabilization of COOH becomes possible by having a Cu atom adjacent to a Au-C primary bond, where it can form a bond with the oxygen end of COOH. As can be seen from high-resolution TEM images and their fast fourier transform ( Fig. 4b and Supplementary Fig. 7 ), the nanoparticles have a uniform phase with d -spacings corresponding to their compositions and the lack of complete Au/Cu atomic ordering, which is in agreement with other characterization methods discussed above. Further, the surface compositions of Au–Cu bimetallic nanoparticles also follow the trend of their bulk compositions, evidenced from XPS spectra ( Fig. 4c and Supplementary Fig. 8 ) at a grazing angle, which is highly surface sensitive. Thus, it is reasonable to assume that both elements are uniformly distributed throughout the particle according to their compositions and that these bimetallic nanoparticles are capable of providing active sites with further COOH stabilization. The electronic effect and geometric effect, operating synergistically here, lead to the observed volcano activity correlation with nanoparticle composition. However, we did not observe a clear trend with the TOR for formate. Formate TOR was rather close in value among the different catalysts ( Supplementary Fig. 6 ). This can also be understood in terms of the change in the binding energy of the intermediates. To produce formate, the active site should be capable of stabilizing both COOH and H, so that there is a high probability of forming a bond between the carbon and the adsorbed proton. However, the relative free energy of adsorbed CO is lower than adsorbed COOH [20] , [21] , [22] . Therefore, COOH is more likely to be converted into CO rather than staying adsorbed as it is ( Supplementary Fig. 9 ). As more Au gets incorporated into Cu, the relative free energy difference between adsorbed COOH and CO narrows [21] . Further, alloy nanoparticles have the capability of further stabilizing COOH due to the geometric effect. Hence, there is higher probability for being adsorbed as COOH. In contrast, the binding strength for H gets weaker as the Au content rises [42] . These two opposing effects lead to HCOO − TOR being relatively unaffected by the compositional shift. Products that require larger number of reaction steps, such as methane or ethylene, diminish significantly even with a slight shift in composition from pure Cu. This might be due to the fact that these products require stabilization of both CO and H. Adsorbed CO is protonated successively to evolve as hydrocarbon species [20] . Cu seems to have the optimum binding strength for both of the adsorbed intermediates to facilitate the conversion. However, as the Au content increases, both intermediates bind weaker, which reduces the TOR and leads to total loss of these products. The use of our unique nanoparticle monolayer not only allows us to carry out the quantitative comparison of the CO 2 reduction activity/selectivity as a function of composition, it also leads to high efficiencies by significantly enhancing mass activities ( Supplementary Fig. 10 and Supplementary Table 2 ). Au 3 Cu, which has the highest mass activity for CO, outperforms conventional Au nanoparticle catalysts [23] by more than an order of magnitude ( Fig. 3b ). There also have been efforts to reduce metal loading by using organometallic catalysts with large enhancements in mass activity [19] . The idea is to significantly reduce the metal loading by having a single metal atom coordinated to organic ligands that can perform the reduction of CO 2 . In the case of Ag, widely known as an efficient catalyst for CO production, this approach led to more than an order-of-magnitude increase in mass activity compared with pure Ag nanoparticles. Our nanoparticle catalyst monolayers, characteristic of efficient loading, can operate at comparable activities to these organometallic catalysts for CO production (even considering the fact that Au is much heavier). The complexity of the reaction is clearly evidenced from the activity trends of Au–Cu bimetallic nanoparticles. The TOR and the product distribution are governed by various intermediates that occur along the reaction pathway. However, we were able to show that this multi-parameter reaction could be described in terms of two effects (as shown in Fig. 4d ), the electronic effect and the geometric effect. From these two factors, one can deduce how the intermediates will interact with the surface of a specific catalyst and hence tune its catalytic activity. To achieve high selectivity towards only CO 2 -reduced products, one should try to mitigate the proton–catalyst interaction (to suppress HER) and at the same time optimize the binding strength of the first few intermediates (COOH and CO) in the pathway by using both effects. However, if the emphasis is on producing products with larger number of electron and proton transfers (that is, methane), the catalyst should be able to stabilize CO even further and allow coupling with the adsorbed proton or hydroxyl groups more efficiently. This might inevitably lead to higher production rates of H 2 , but if the atomic configuration on the active site prohibits proton–proton coupling, one might be able to achieve higher selectivity even for more complex products as well. In the design of a CO 2 reduction catalyst, one should carefully balance how these two effects determine the interaction of intermediates with the catalyst so as to achieve better activity and selectivity. We have used monodisperse Au–Cu bimetallic nanoparticles in a unique platform to understand the trends of their fundamental activity for CO 2 reduction. With its connection to the electronic structure and the local atomic environment, we could understand their catalytic activity systematically and have determined the factors that allow us to simplify the picture of the overall CO 2 reduction. Further, our unique monolayer platform enabled us to measure mass activities significantly higher than catalysts structured by more conventional means. With the principles of catalyst design established, coupled with exceptional structuring of active sites, we believe unprecedented improvements in electrochemical CO 2 reduction will be eventually fulfilled that will allow our goals of a sustainable energy society to finally become a reality. Nanoparticle synthesis Au–Cu bimetallic nanoparticles were synthesized via the co-reduction of metal precursors. For the Au–Cu bimetallic nanoparticle (1:1 ratio), first, 1-octadecene (Sigma Aldrich) was heated to 130 °C for 30 min under nitrogen atmosphere. Next, 2 mmol of oleic acid (Sigma Aldrich), 2 mmol of oleylamine (Sigma Aldrich), 0.5 mmol of gold acetate (Alfa Aesar), 0.5 mmol of copper acetate (Sigma Aldrich) and 4 mmol of 1,2-hexadecanediol (Sigma Aldrich) were added. Under the inert atmosphere, the mixture was heated to 200 °C and kept at that temperature for 2 h while stirring. Afterwards, it was further heated to 280 °C for 1 h. Then, the reaction was stopped by cooling it down to room temperature. Ethanol was added to the mixture to precipitate the synthesized nanoparticles and was washed several times with hexane and ethanol by centrifugation. For other compositions, the ratio of gold acetate to copper acetate was modified. The bimetallic nanoparticles showed significant stability against oxidation in ambient atmosphere and we kept the as-made nanoparticles in hexane. In the case of a pure Cu nanoparticle, synthetic procedures with tetradecylphosphonic acid (Sigma Aldrich) were followed instead, to inhibit its full conversion to Cu 2 O [28] . The nanoparticles were characterized by XRD (Bruker D8), TEM (Hitachi H-7650, JEOL 2100F), ultraviolet-visible spectroscopy (Vernier) and energy-dispersive X-ray spectroscopy (EDAX). Monolayer assembly Nanoparticle assembly was conducted with methods modified from the previous report [38] . In the case of AuCu, 1.8 ml of AuCu nanoparticle solution (1 mg ml −1 in hexane) was added to a solution mixture of 5 ml of hexane and 3 ml of toluene. Then, 600~700 μl of the diluted nanoparticle solution was carefully spread on top of the water surface inside a custom-designed glass trough. The nanoparticle solution was left to evaporate through the opening at one end of the trough. After the solvent mixture dried, a large portion of the glass trough was covered with nanoparticle monolayer films. The monolayer films were transferred onto various substrates by the Langmuir–Schaefer method for further experiments. The transferred monolayers were imaged by TEM and scanning electron microscopy (JEOL JSM-6340F). XPS (PHI 5400) measurements were carried out on the monolayers to identify their electronic structure and surface composition. Using an Al Kα source, with the pressure inside the chamber maintained below ~4 × 10 −9 Torr, the spectra were collected at a pass energy of 17.9 eV. All the spectra collected were corrected using a Shirley background. Compositions were determined by considering the atomic sensitivity factors. Centre of gravity calculation for the valence band spectra is conducted as in the range of 0~−9.0 eV, where N(ε) is the density of states. Electrochemical measurement All electrochemical measurements were carried out in our customized electrochemical setup. The cell has two compartments that are separated by an anion exchange membrane (Selemion AMV). Pt was used as a counter electrode and Ag/AgCl (1 M KCl) as a reference electrode. The nanoparticle monolayer on glassy carbon substrate was transferred inside the cell to test its CO 2 reduction activity. Electrolyte (33 ml in the working compartment with gas headspace ~7 ml) used was 0.1 M KHCO 3 made from de-ionized water (Ricca Chemical). Before every measurement, the working electrode compartment was purged with CO 2 (Praxair, 5.0 Ultra high purity) for 30 min at a flow rate of 30 ml min −1 . All the electrolysis was conducted at room temperature and 1 atm CO 2 with pH of the electrolyte at 6.8. During chronoamperometry, effluent gas from the cell went through the sampling loop of a gas chromatograph (SRI) and was analysed in 20 min intervals to determine the concentration of gas products. The gas chromatograph was equipped with a molecular sieve 13X and hayesep D column with Ar (Praxair, 5.0 Ultra high purity) flowing as a carrier gas. The separated gas products were analysed by a thermal conductivity detector (for H 2 ) and a flame ionization detector (for CO and hydrocarbons). Liquid products were analysed afterwards by quantitative NMR (Bruker AV-500) using dimethyl sulphoxide as an internal standard. Solvent presaturation technique was implemented to suppress the water peak. The concentration of liquid products was determined by the standard curves made from various known concentrations (0.05, 0.1, 0.5 and 1 mM) of chemicals purchased. FEs were calculated from the amount of charge passed to produce each product divided by the total charge passed at a specific time or during the overall run (for liquid products). Relative turnover was compared based on the partial current density for each product. Mass activities were calculated based on the overall mass of Au and Cu for each nanoparticle and the mass loading was determined assuming complete hexagonal packing on the substrate. Each measurement was conducted three times to check the consistency of our experiments. Electrochemical data presented here are the average values out of these multiple measurements. How to cite this article: Kim, D. et al . Synergistic geometric and electronic effects for electrochemical reduction of carbon dioxide using gold–copper bimetallic nanoparticles. Nat. Commun. 5:4948 doi: 10.1038/ncomms5948 (2014).